DAF-16/FOXO requires Protein Phosphatase 4 to initiate transcription of stress resistance and longevity promoting genes In C. elegans, the conserved transcription factor DAF-16/FOXO is a powerful aging regulator, relaying dire conditions into expression of stress resistance and longevity promoting genes. For some of these functions, including low insulin/IGF signaling (IIS), DAF-16 depends on the protein SMK-1/SMEK, but how SMK-1 exerts this role has remained unknown. We show that SMK-1 functions as part of a specific Protein Phosphatase 4 complex (PP4 SMK-1 ). Loss of PP4 SMK-1 hinders transcriptional initiation at several DAF-16-activated genes, predominantly by impairing RNA polymerase II recruitment to their promoters. Search for the relevant substrate of PP4 SMK-1 by phosphoproteomics identified the conserved transcriptional regulator SPT-5/SUPT5H, whose knockdown phenocopies the loss of PP4 SMK-1 . Phosphoregulation of SPT-5 is known to control transcriptional events such as elongation and termination. Here we also show that transcription initiating events are influenced by the phosphorylation status of SPT-5, particularly at DAF-16 target genes where transcriptional initiation appears rate limiting, rendering PP4 SMK-1 crucial for many of DAF-16’s physiological roles. Insulin/IGF-like signaling (IIS) is one of the most prominent aging-regulatory pathways. Conserved from worms to mammals [1] , [2] , it has critical roles in the regulation of metabolism, reproduction, stress resistance, and longevity [3] , [4] . In particular the stress resistance and longevity phenotypes are controlled through a conserved downstream transcription factor called DAF-16/FOXO. Under normal conditions, IIS is active and phosphorylates DAF-16 via AKT and SGK kinases, leading to the sequestration of DAF-16 in the cytoplasm through interaction with 14-3-3, away from its target genes. However, under dire conditions—those leading to low IIS in particular—phosphorylation is reduced, allowing DAF-16 to translocate into the nucleus. There it binds to the promoters and regulates transcription of its target genes, predominantly inducing genes that contribute to stress response mechanisms and promote longevity [5] , [6] . Although nuclear translocation of DAF-16 is a prerequisite, it is not sufficient for DAF-16 to regulate its target genes [7] . Additional regulators and cofactors are needed. One of the most powerful positive regulators of DAF-16, the conserved protein SMK-1/SMEK, was described already a decade ago [8] . Under low IIS, SMK-1 is required for DAF-16-driven longevity and the resistance to oxidative stress, to ultraviolet (UV) irradiation, and to pathogens. Interestingly though, it is not required for DAF-16 to promote thermotolerance, to promote dauer formation, or to delay reproduction [8] . This suggests that SMK-1 genetically interacts with DAF-16 but regulates only parts of its functions, likely by influencing the expression of only a specific subset of its target genes. Despite this prior work and the interesting phenotypes observed, the mechanism by which SMK-1 would influence gene expression has remained unknown. Here we show that SMK-1 acts as part of a specific Protein Phosphatase 4 complex, PP4 SMK-1 , which binds and dephosphorylates the transcriptional regulator SPT-5. Under low IIS, this dephosphorylation of SPT-5 promotes transcription initiating events, in particular RNA Pol II (Pol II) recruitment  at several DAF-16 target genes, and thereby promotes a large part of DAF-16’s functions. SMK-1 is part of a nuclear Protein Phosphatase 4 complex To gain insight into the mechanism by which SMK-1 promotes DAF-16 functions, we sought to identify proteins bound to SMK-1. We grew Caenorhabditis elegans expressing SMK-1::mCherry to large quantity, lysed them, and conducted an immunoprecipitation (IP) using anti-mCherry antibody. The precipitate was then analyzed by silver staining (Fig. 1a ) and tandem mass spectrometry (MS/MS, Fig. 1b ). By this approach, we found 16 proteins that co-purified with SMK-1::mCherry (Fig. 1b, c , see Supplementary Table 2 for an independent repeat). 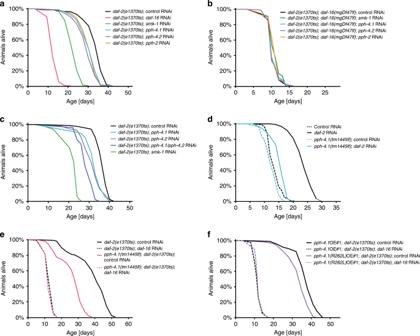Fig. 2: SMK-1 promotes the DAF-16-mediated longevity induced by low IIS as part of PP4SMK-1. Lifespan phenotypes caused by loss ofdaf-16or specific PP4 subunits in various genetic backgrounds. Animals of indicated genotypes were grown from the L1 stage on the indicated RNAi bacteria at 15 °C. At the L4 stage the animals were shifted to 25 °C to fully inactivatedaf-2(e1370ts)and their lifespan was monitored. All strains used ina–charbored theeri-1(mg366ts)mutation to yield better knockdown efficiencies51.aIndividual knockdown ofdaf-16or any of the PP4SMK-1subunits shortened the lifespan ofdaf-2(e1370ts)mutant animals.bAll these phenotypes were abolished indaf-16(mgDf47lf)null mutant animals.cCombined knockdown of the catalytic PP4SMK-1subunit paralogspph-4.1andpph-4.2enhanced the lifespan-shortening effects of their individual knockdowns indaf-2(e1370ts)mutant animals.d,eThepph-4.1(tm1445lf)null mutation strongly impaired the longevity of low IIS animals in adaf-16-dependent manner, too.fLifespan analyses ofdaf-2(e1370ts)mutant animals ectopically expressing either catalytically active PPH-4.1 or catalytic dead PPH-4.1(R262L). Expression of the catalytically dead PPH-4.1(R262L) specifically impaired the longevity ofdaf-2(e1370ts)mutant animals. For detailed statistics see Supplementary Table4. Source data are provided as a Source Data file. The most abundant of these were subunits of Protein Phosphatase 4 (PP4); namely the catalytic subunits PPH-4.1 and PPH-4.2, and the regulatory subunit PPFR-2 (Fig. 1b, c ). According to previous work in yeast and mammals, PP4 complexes exist in different defined subunit compositions. Each complex contains a catalytic subunit of PP4, of which the closest C. elegans orthologs are PPH-4.1 and PPH-4.2, and it contains a selection of four regulatory subunits, which help to target PP4 to its substrates [9] , [10] , [11] . Closest C. elegans orthologs to three of these regulatory subunits are PPFR-1, PPFR-2, and PPFR-4. Strikingly, closest ortholog to the fourth regulatory subunit is SMK-1. Together with our IP–MS/MS data, this suggests that SMK-1 is actually a regulatory subunit of a specific PP4 complex in C. elegans , hereafter referred to as PP4 SMK-1 . This complex has a unique subunit composition, containing either of the catalytic subunits and the regulatory subunits SMK-1 and PPFR-2, but not PPFR-1 or PPFR-4 (see also Fig. 1c ). Next, we sought to confirm this result by independent IP–MS/MS experiments, using a different epitope tag on SMK-1 and a different affinity matrix (SMK-1::GFP and GFP-Trap, respectively). Given that SMK-1 is required for DAF-16 functions when IIS activity is low but not when it is high [8] , we further tested in this experiment whether the incorporation of SMK-1 into the PP4 SMK-1 complex is IIS-dependent, by conducting the IPs from either daf-2(e1370) (a mutant of the insulin/IGF receptor, resulting in low IIS) or daf-18(mg198) (a mutant of PTEN, resulting in high IIS) animals. We confirmed the existence and composition of the PP4 SMK-1 complex and found that the formation of this complex was not affected by IIS activity (Supplementary Table 3 ). 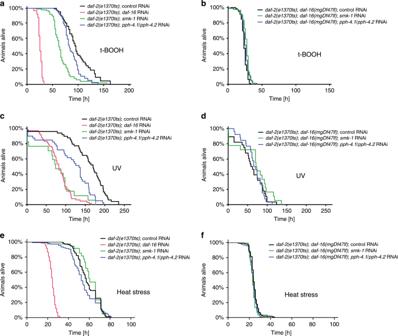Fig. 3: Under low IIS, PP4SMK-1is required for DAF-16-mediated resistance to oxidative stress and UV. Stress survival phenotypes caused by loss ofdaf-16or PP4SMK-1in various genetic backgrounds. Animals of indicated genotypes were grown at 15 °C from the L1 stage on the indicated RNAi bacteria. At the L4 stage the temperature was shifted to 25 °C to fully inactivatedaf-2(e1370ts). On day 2 adulthood, animals were then transferred to 6 mM tBOOH containing RNAi plates (oxidative stress), exposed to 1500 J/m2UV light (UV stress), or shifted to 32 °C (heat stress). All strains used in in this figure harbored theeri-1(mg366ts)mutation to yield better knockdown efficiencies51.a,cLoss of PP4SMK-1, either by knockdown of SMK-1 or double knockdown of PPH-4.1/PPH-4.2, impaired the enhanced survival ofdaf-2(e1370ts)mutant animals that were exposed to oxidative stress (a) or UV stress (c).b,dThese phenotypes were abolished in the absence ofdaf-16.e,fIn contrast to oxidative stress and UV stress, loss of these PP4SMK-1subunits did not impair the enhanced survival ofdaf-2(e1370ts)mutant animals exposed to heat stress. For detailed statistics see Supplementary Table4. Source data are provided as a Source Data file. As a final demonstration of how readily SMK-1 incorporates into PP4 SMK-1 complexes in vivo, we expressed a minimal C. elegans PP4 SMK-1 complex comprised of SMK-1::HA 3 , PPFR-2, and PPH-4.1::TAP in Saccharomyces cerevisiae , purified PPH-4.1-TAP by IgG pulldown, and then detected SMK-1::HA 3 by western blotting. SMK-1::HA 3 specifically co-purified with PPH-4.1::TAP (Supplementary Fig. 9d ). Fig. 1: SMK-1 is part of a globally expressed nuclear Protein Phosphatase 4 complex. a SDS-PAGE and silver staining analysis of an anti-mCherry immunoprecipitation from whole-animal lysates of C. elegans expressing SMK-1::mCherry. Animals expressing no transgene were used as negative control. b List of the proteins identified in the purification from a , as determined by mass spectrometry (LC–MS/MS). Only proteins identified by at least two unique peptides are shown. See also Supplementary Table 2 for an independent repeat of this experiment. c Model illustrating the composition of the specific Protein Phosphatase 4 complex (PP4 SMK-1 ) that co-purified with SMK-1, next to other implicated PP4 subunits not found in this complex. d Localization studies of DAF-16::GFP, SMK-1::GFP, and PPH-4.1::GFP in wild type and in daf-2(e1370ts) mutant animals. Worms were grown from the L1 stage at 15 °C, then shifted to 25 °C at the L2/L3 stage. After 16 h the GFP signal was recorded in L4 animals (yellow scale bar: 100 µm). The higher magnification images for PPH-4.1::GFP show head regions. Arrows are highlighting the partial nuclear accumulation of PPH-4.1 in both wild type and daf-2(e1370ts) animals (white scale bar: 20 µm). Full size image A surprising observation in these SMK-1 IPs was the prominent presence of the phosphatase subunit PAA-1 (Fig. 1b, c , Supplementary Tables 2 , 3 ). PAA-1 is a well-established scaffold subunit of Protein Phosphatase 2A (PP2A) complexes [12] that had not been found in PP4 complexes before. Our data suggests that, at least in C. elegans , PAA-1 may also be part of PP4 complexes, or alternatively that SMK-1 may be part not only of PP4 SMK-1 but also a PP2A-related complex. Future studies will have to evaluate this. Next, we were interested in the localization of the PP4 SMK-1 complex, to get an indication of the tissues and cellular compartments, in which the complex regulates DAF-16 function under low IIS. We studied wild type and daf-2(e1370) animals expressing either SMK-1::GFP or PPH-4.1::GFP under their endogenous promoters. Animals expressing DAF-16::GFP served as additional control. We found that similar to DAF-16::GFP also SMK-1::GFP and PPH-4.1::GFP were globally expressed (Fig. 1d , Supplementary Fig. 1 , see also [8] , [13] ). Within cells, SMK-1::GFP localized strictly to the nucleus, while PPH-4.1::GFP could be seen in both the nucleus and cytoplasm (Fig. 1d , Supplementary Fig. 1 ). Expression pattern and subcellular localization of SMK-1::GFP and PPH-4.1::GFP were not affected by changes in IIS activity (Fig. 1d , Supplementary Fig. 1 ). This data showed that under low IIS the PP4 SMK-1 complex has the opportunity to form in all tissues, and the intracellular localization patterns of its subunits suggest that the complex resides and exerts its functions in the nucleus. PP4 SMK-1 is required for DAF-16 to promote longevity In light of this complex formation, we tested whether SMK-1 contributes to DAF-16’s functions as part of PP4 SMK-1 —in particular through the complex’s catalytic activity. First, we explored the role of PP4 SMK-1 for lifespan regulation by DAF-16. We began by individually knocking down all PP4 SMK-1 complex subunits by RNAi, either in daf-2 mutant animals, which are long-lived due to constitutive DAF-16 activation, or in daf-2; daf-16 mutant animals, where this DAF-16-driven effect is absent. Consistent with SMK-1 acting as part of PP4 SMK-1 , smk-1 as well as pph-4.1 , pph-4.2 and ppfr-2 were all required for full lifespan extension in daf-2 mutant animals (Fig. 2a ). Importantly, their influence on lifespan was completely dependent on the presence of daf-16 (Fig. 2b ). Next, we wanted to compare the ability of PP4 SMK-1 versus other PP4 complexes to promote DAF-16 functions. For this we extended the previous experiment to include knockdowns of ppfr-1 and ppfr-4 —two PP4 subunits that we found to be absent from PP4 SMK-1 (Fig. 1b, c ). Consistent with PP4 SMK-1 being the preferred PP4 configuration to regulate DAF-16 functions, loss of ppfr-1 had no effect on lifespan (Supplementary Fig. 2a, b ). And although loss of ppfr-4 shortened the lifespan of daf-2 animals, it did so in a manner independent of daf-16 (Supplementary Fig. 2a, b ). Fig. 2: SMK-1 promotes the DAF-16-mediated longevity induced by low IIS as part of PP4 SMK-1 . Lifespan phenotypes caused by loss of daf-16 or specific PP4 subunits in various genetic backgrounds. Animals of indicated genotypes were grown from the L1 stage on the indicated RNAi bacteria at 15 °C. At the L4 stage the animals were shifted to 25 °C to fully inactivate daf-2(e1370ts) and their lifespan was monitored. All strains used in a – c harbored the eri-1(mg366ts) mutation to yield better knockdown efficiencies [51] . a Individual knockdown of daf-16 or any of the PP4 SMK-1 subunits shortened the lifespan of daf-2(e1370ts) mutant animals. b All these phenotypes were abolished in daf-16(mgDf47lf) null mutant animals. c Combined knockdown of the catalytic PP4 SMK-1 subunit paralogs pph-4.1 and pph-4.2 enhanced the lifespan-shortening effects of their individual knockdowns in daf-2(e1370ts) mutant animals. d , e The pph-4.1(tm1445lf) null mutation strongly impaired the longevity of low IIS animals in a daf-16 -dependent manner, too. f Lifespan analyses of daf-2(e1370ts) mutant animals ectopically expressing either catalytically active PPH-4.1 or catalytic dead PPH-4.1(R262L). Expression of the catalytically dead PPH-4.1(R262L) specifically impaired the longevity of daf-2(e1370ts) mutant animals. For detailed statistics see Supplementary Table 4 . 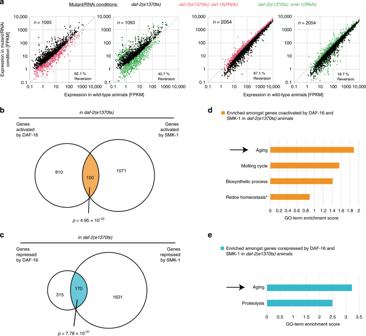Fig. 4: PP4SMK-1is required for a substantial part of the DAF-16-mediated gene expression changes induced by low IIS. daf-2(e1370ts)mutantC. eleganswere grown from the L1 stage on either control,daf-16, orsmk-1RNAi bacteria. At the L4 stage, animals were shifted for 16 h to 25 °C, then harvested, and their transcriptomes determined by mRNA-seq. All strains used in in this figure harbored theeri-1(mg366ts)mutation to yield better knockdown efficiencies51.aSimilar todaf-16loss,smk-1loss also suppresses many of the gene expression changes that occur under low IIS. The scatter plots on the left show the genes significantly upregulated and the scatter plots on the right show the genes significantly downregulated indaf-2(e1370ts)compared with wild type animals.b,cVenn diagrams illustrate the number of genes significantly regulated by DAF-16 or SMK-1 indaf-2(e1370ts)mutant animals as well as their overlap.d,eFunctional enrichment analyses, conducted on the co-activated and co-repressed genes shown inbandc. Only significant enrichments are shown (DAVID scores ≥1.3, the symbol asterisk indicates that this term was still amongst the four most enriched GO-terms and relevant in the context of aging and stress responses, but it had a score below the significance threshold). Arrows highlight the GO-term “aging”, which turned out to be the most enriched in both analyses. Source data are provided as a Source Data file. Full size image In Fig. 2a , RNAi of pph-4.1 or pph-4.2 had a lesser effect on DAF-16-driven longevity than RNAi of smk-1 . We attributed this to a possible redundancy of these two PP4 catalytic subunits. To test this, we conducted double-RNAi experiments targeting pph-4.1 and pph-4.2 together. Indeed, combined knockdown of both catalytic subunits led to additive suppression of longevity in daf-2 animals, to an extent now more comparable to smk-1 RNAi (Fig. 2c ). Again, these lifespan phenotypes were dependent on daf-16 , as illustrated by conducting the same knockdowns in wild type (Supplementary Fig. 2c ) or daf-2; daf-16 mutant animals (Supplementary Fig. 2d ). We then validated the phenotypes obtained from knockdown of the PP4 SMK-1 catalytic subunits using a loss-of-function allele of pph-4.1 , pph-4.1(tm1445) . This allele lacks exons 3 and 4 of pph-4.1 , which contain the active site of the enzyme. Consistent with our RNAi data, this allele also specifically suppressed the longevity of daf-2 mutant animals, while it had little effect in wild type and no effect in daf-2; daf-16 mutant animals (Fig. 2d, e ). So far, our data was consistent with SMK-1 and PPH-4.1/4.2 each affecting lifespan as part of the PP4 SMK-1 complex, acting through the same genetic pathway. If this were true, then combined depletion of smk-1 and pph-4.1/4.2 should lead to largely nonadditive phenotypes. We tested this by lifespan assays in daf-2 mutant animals, confirming that this was indeed the case (Supplementary Fig. 2e ). Finally, we tested if it is truly the catalytic activity rather than structural properties of PP4 SMK-1 that promote DAF-16 functions. We created transgenic lines overexpressing either wild type pph-4.1 or an allele encoding an R262L mutant form of PPH-4.1, which has been shown to be catalytically inactive by studies in C. elegans and mammals [14] , [15] . Consistent with the importance of the catalytic activity of PP4 SMK-1 , overexpression of the catalytic dead form of PPH-4.1 led to partial suppression of longevity in daf-2 mutant animals (Fig. 2f , Supplementary Fig. 2f ), and this lifespan-shortening effect was lost upon knockdown of daf-16 (Fig. 2f , Supplementary Fig. 2f ). We conclude that SMK-1 acts as part of a specific PP4 complex and uses its catalytic activity to promote DAF-16 functions, as shown here for DAF-16-driven longevity under low IIS. PP4 SMK-1 promotes only some DAF-16-driven stress responses Much of the DAF-16-driven longevity in daf-2 mutant animals can be attributed to improved stress responses [6] . Consistently, a previous study had shown that SMK-1 was required for the daf-16 -dependent improved resistance of daf-2 animals to oxidative stress and UV irradiation [8] . Notably though, SMK-1 showed surprising specificity in mediating these phenotypes, as it did not affect the daf-16 -dependent increased resistance to for example heat stress in these animals [8] . We now tested, if PP4 SMK-1 confers stress resistance with similar specificity. For this we knocked down the catalytic subunits, pph-4.1 and pph-4.2 , by combined RNAi in either daf-2 or daf-2 ; daf-16 mutant animals and exposed them to either 1500 J/m 2 UV irradiation or shifted them to 6 mM tert-butyl hydroperoxide (tBOOH; oxidative stress) or to 32 °C (heat stress) at day 2 of adulthood. Survival under these stresses was determined using a lifespan scoring machine [16] , to obtain data of particularly high resolution. We found that just like RNAi against smk-1 , RNAi against pph-4.1/pph-4.2 also led to reduced resistance to tBOOH and UV irradiation but not to heat (Fig. 3a, c, e ). Furthermore, consistent with these being daf-16 -dependent effects, these phenotypes were reduced in wild type animals when daf-16 activity is reduced (Supplementary Fig. 3 ), and were entirely absent in daf-16 null mutant animals (Fig. 3b, d, f ). Fig. 3: Under low IIS, PP4 SMK-1 is required for DAF-16-mediated resistance to oxidative stress and UV. Stress survival phenotypes caused by loss of daf-16 or PP4 SMK-1 in various genetic backgrounds. Animals of indicated genotypes were grown at 15 °C from the L1 stage on the indicated RNAi bacteria. At the L4 stage the temperature was shifted to 25 °C to fully inactivate daf-2(e1370ts) . On day 2 adulthood, animals were then transferred to 6 mM tBOOH containing RNAi plates (oxidative stress), exposed to 1500 J/m 2 UV light (UV stress), or shifted to 32 °C (heat stress). All strains used in in this figure harbored the eri-1(mg366ts) mutation to yield better knockdown efficiencies [51] . a , c Loss of PP4 SMK-1 , either by knockdown of SMK-1 or double knockdown of PPH-4.1/PPH-4.2, impaired the enhanced survival of daf-2(e1370ts) mutant animals that were exposed to oxidative stress ( a ) or UV stress ( c ). b , d These phenotypes were abolished in the absence of daf-16 . e , f In contrast to oxidative stress and UV stress, loss of these PP4 SMK-1 subunits did not impair the enhanced survival of daf-2(e1370ts) mutant animals exposed to heat stress. For detailed statistics see Supplementary Table 4 . Source data are provided as a Source Data file. Full size image These data illustrate that SMK-1’s roles in promoting stress resistance under low IIS also rely on the catalytic subunits of PP4 SMK-1 ; and we could confirm the prior observation that SMK-1, and now PP4 SMK-1 , selectively help DAF-16 to confer a subset of its stress responses, e.g. resistance to oxidative stress and UV but not heat stress. PP4 SMK-1 influence expression of many DAF-16 target genes Given that PP4 SMK-1 is required for many of DAF-16’s functions under low IIS, and because DAF-16 is a transcription factor, we wondered whether PP4 SMK-1 acts by influencing the expression of DAF-16-regulated genes. We conducted mRNA-seq experiments using either wild type or daf-2 mutant C. elegans . The animals were treated with either control, daf-16 , or smk-1 RNAi from the L1 stage and their mRNA sequenced at young adulthood. From the resulting dataset, we first determined the genes differentially expressed by the reduced IIS in daf-2 mutant animals, identifying 1093 upregulated and 2054 downregulated genes (Fig. 4a ). These gene expression changes were consistent with previous work [17] (Supplementary Table 9 ). Next we asked how these differentially expressed genes are affected by RNAi against daf-16 or smk-1 in daf-2 mutant animals. Most of the gene expression changes that occur in daf-2 mutant animals are known to be mediated by DAF-16 [6] , [17] . In agreement with this prior work, RNAi of daf-16 suppressed 62.1% of the gene activation and 87.1% of the gene repression events in daf-2 mutant animals (Fig. 4a , Supplementary Table 9 ). RNAi of smk-1 also suppressed many of these gene expression changes, namely 40.7% and 18.7%, respectively (Fig. 4a ). These findings were consistent with PP4 SMK-1 indeed influencing the lifespan extending and largely DAF-16-induced gene expression changes under low IIS. Next we determined which actual genes were regulated by DAF-16 or SMK-1 under low IIS and which genes were common targets of both. As expected from the results in Fig. 4a , we found significant overlap amongst the genes that were activated or amongst the genes that were repressed by DAF-16 and SMK-1 ( p = 4.95 × 10 −22 and p = 7.78 × 10 −51 , respectively; Fig. 4b, c ). And consistent with both DAF-16 and SMK-1 being required for the longevity under low IIS, we found these co-regulated genes to be enriched for genes related to aging (based on GO-term enrichment analyses, Fig. 4d, e ). Fig. 4: PP4 SMK-1 is required for a substantial part of the DAF-16-mediated gene expression changes induced by low IIS. daf-2(e1370ts) mutant C. elegans were grown from the L1 stage on either control, daf-16 , or smk-1 RNAi bacteria. At the L4 stage, animals were shifted for 16 h to 25 °C, then harvested, and their transcriptomes determined by mRNA-seq. All strains used in in this figure harbored the eri-1(mg366ts) mutation to yield better knockdown efficiencies [51] . a Similar to daf-16 loss, smk-1 loss also suppresses many of the gene expression changes that occur under low IIS. The scatter plots on the left show the genes significantly upregulated and the scatter plots on the right show the genes significantly downregulated in daf-2(e1370ts) compared with wild type animals. b , c Venn diagrams illustrate the number of genes significantly regulated by DAF-16 or SMK-1 in daf-2(e1370ts) mutant animals as well as their overlap. d , e Functional enrichment analyses, conducted on the co-activated and co-repressed genes shown in b and c . Only significant enrichments are shown (DAVID scores ≥1.3, the symbol asterisk indicates that this term was still amongst the four most enriched GO-terms and relevant in the context of aging and stress responses, but it had a score below the significance threshold). Arrows highlight the GO-term “aging”, which turned out to be the most enriched in both analyses. Full size image Taken together, PP4 SMK-1 is required for DAF-16 to properly regulate a subset of its target genes—many of which are aging related. PP4 SMK-1 barely affects DAF-16 activation and DNA binding Having established that PP4 SMK-1 is important for many DAF-16 functions under low IIS, presumably by helping it to regulate aging-related target genes, we wondered how this function arises. Between the initial DAF-16-activating stimulus of low IIS activity and the successful regulation of target genes resides a long series of events. At which level of this cascade does PP4 SMK-1 act? First, we studied the kinetics of nuclear entry and exit of DAF-16 upon inactivation and reactivation of the temperature-sensitive daf-2(e1370) allele, respectively (Supplementary Fig. 4a ). Previous work only comparing translocation endpoints had found no impact of SMK-1 on the nuclear translocation of DAF-16 [8] . Consistently, we observed no difference in the endpoints of our nuclear entry and nuclear exit time courses (Supplementary Figs. 4b, c , and 5 ). Only when we followed the kinetics of nuclear translocation we observed that knockdown of smk-1 led to a mild delay, particularly in the entry of DAF-16 upon daf-2 inactivation (Supplementary Figs. 4b, c and 5 ). However, we interpret this phenotype as very moderate and hence unlikely to explain the strong impact of PP4 SMK-1 on DAF-16 functions. Upon nuclear entry of DAF-16, it next needs to bind to its target promoters (Supplementary Fig. 4a ). To see if this is influenced by PP4 SMK-1 we determined the genome-wide binding of DAF-16 to its target promoters in the presence or absence of SMK-1. We used daf-2 mutant animals expressing DAF-16::GFP, treated them with either control or smk-1 RNAi, and then subjected them to chromatin immunoprecipitation (ChIP)-seq analysis using an anti-GFP antibody. Looking across 2824 DAF-16 binding sites described in previous work [18] , we found no significant change in the binding of DAF-16 to its target regions ( p = 0.152; Supplementary Fig. 4d ; see also Supplementary Fig. 4e for examples of individual genes contributing to Supplementary Fig. 4d ). In summary, absence of SMK-1 led to only a slight delay in DAF-16 nuclear entry and no significant change in the binding of DAF-16 to its target promoters. We therefore conclude that PP4 SMK-1 ’s main impact on DAF-16 function should occur yet further downstream. PP4 SMK-1 promotes transcription initiating events DAF-16 is predominantly a transcriptional activator [17] . Thus, upon binding its target promoters the next important downstream steps should be: (1) the recruitment of RNA Polymerase II (Pol II) to the promoters; (2) promoter clearance, which causes Pol II to leave the promoter region and move into the gene body where it often will pause around the +50 position (promoter-proximal pausing) [19] , [20] ; (3) transcriptional elongation, during which Pol II moves beyond the pause site and transcribes the entire gene (Fig. 5a ). To evaluate these steps we used daf-2 mutant animals, subjected them to either control or smk-1 RNAi, and then determined the genome-wide distribution of Pol II on chromatin by ChIP-seq using an antibody against the large subunit of Pol II, AMA-1. Strikingly, while Pol II recruitment was unaffected by smk-1 RNAi when looking cumulatively at all promoter regions genome-wide ( p = 0.796), we saw a substantial reduction in Pol II recruitment to promoters whose downstream genes would both be activated by DAF-16 and depend on SMK-1 for their activation (genes co-activated by DAF-16 and SMK-1 according to Fig. 4b ) ( p = 0.012; Fig. 5b , see left panels of Supplementary Fig. 6 for examples of genes that exhibit this phenotype). Fig. 5: PP4 SMK-1 is required for transcription initiating events at the genes co-activated by DAF-16 and SMK-1. a Schematic of the key steps that lead from DAF-16’s binding to promoter regions to the eventual transcription of the downstream genes. b – d ChIP-seq analysis of RNA Pol II under low IIS. daf-2(e1370ts) mutant animals were synchronized and grown from the L1 stage on either control or smk-1 RNAi bacteria. At the L4 stage, animals were shifted to 25 °C. After an additional 16 h, animals were harvested and ChIP-seq analysis was conducted, using antibodies recognizing RNA Pol II, either in any modification state ( b , c ) or specifically RNA Pol II that was phosphorylated at Ser5 of its CTD ( d ). Average read densities across TSS regions of the indicated gene sets are shown. p values indicate the significance of read density differences in the grayed regions (−600 to +600 around the TSSs) between control and smk-1 RNAi treated animals. Source data underlying Fig. 5 b, d are provided as a Source Data file. Full size image Besides this apparent phenotype, we also noted an unexpected distribution of Pol II at these promoters. When we looked cumulatively at the regions around transcriptional start sites (TSSs) genome-wide, most Pol II had already undergone transcriptional initiation and localized to the pause site in the gene body (Fig. 5c ). A similar distribution of Pol II could be found when looking cumulatively at all genes activated by DAF-16 (Fig. 5c ). However, at the genes co-activated by DAF-16 and SMK-1, the distribution of Pol II was noticeably wider and a substantial amount of Pol II localized upstream of the TSS (Fig. 5c , see red arrow). We believe that this Pol II has been recruited to promoters but not fully undergone promoter clearance yet, which may indicate that the events of transcriptional initiation at DAF-16/SMK-1-co-activated genes occur slower and hence may be particularly rate limiting for their transcription [21] . Upon smk-1 RNAi, presence of Pol II upstream of the TSS was even more pronounced (Fig. 5b ), which would be consistent with SMK-1 promoting not only Pol II recruitment but also promoter clearance. However, we remain uncertain of this phenotype as it was difficult to recapitulate on the level of individual genes (see right panels of Supplementary Fig. 6 for example genes). To further test our notion of transcription initiating events being impaired, we repeated our ChIP-seq experiments using an antibody that detects only initiating Pol II, which is phosphorylated at the Ser5 position within the repeats of its C-terminal domain (CTD) [22] , [23] . Indeed, we found significantly less initiating Pol II in the TSS regions of DAF-16/SMK-1-co-activated genes (Fig. 5d ). Finally, we investigated if PP4 SMK-1 influences Pol II pausing, pause release or transcriptional elongation. A good indicator for defects in these processes are changes in the pausing index (the ratio of the average read densities of paused to elongating Pol II), as it can be derived from Pol II ChIP-seq data [24] . Calculating this index for DAF-16/SMK-1-co-activated genes under low IIS we found no impact of smk-1 RNAi on the pausing index (Supplementary Table 6 ), suggesting that PP4 SMK-1 had no direct role in Pol II pausing, pause release or transcriptional elongation. We conclude that PP4 SMK-1 is required for transcriptional initiation, predominantly by promoting efficient Pol II recruitment at a subset of DAF-16-activated target genes, and that these are genes whose expression may particularly depend on transcriptional initiation as a rate limiting step. 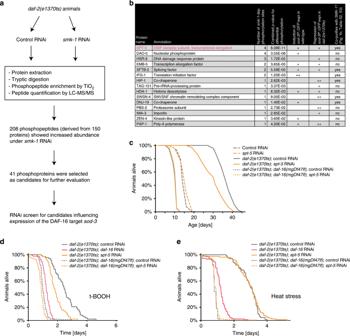Fig. 6: PP4SMK-1promotes DAF-16’s functions under low IIS by dephosphorylating SPT-5. Identification of the relevant PP4SMK-1substrate by unbiased phosphoproteomics and functional evaluation of the emerging candidates.aWorkflow of the phosphoproteomics approach to identify PP4SMK-1substrate candidates, followed by their functional evaluation through RNAi screening using asod-3P::GFPreporter in either wild type ordaf-2(e1370ts)backgrounds.bResults from the approach shown undera. The table is limited to proteins that were found significantly more phosphorylated uponsmk-1RNAi and that additionally affected expression ofsod-3, i.e., bysod-3induction in wild type or the repression ofsod-3expression indaf-2(e1370ts)mutant animals. The table is ranked by the significance (pvalue) of the increased phosphorylation observed uponsmk-1RNAi. SPT-5 is highlighted in red as being the top-ranked candidate from this prioritization approach.c–eLoss of SPT-5 phenocopied the stress resistance and lifespan phenotypes caused by loss of SMK-1. All strains used in in this figure harbored theeri-1(mg366ts)mutation to yield better knockdown efficiencies51. Wild type,daf-2(e1370ts), ordaf-16(mgDf47lf);daf-2(e1370ts)mutant animals were grown from the L4 stage on either control orspt-5RNAi bacteria at 25°C. Animals remained either untreated (c), or were grown until day 2 of adulthood and then transferred to either 6 mM tBOOH containing RNAi plates (oxidative stress) (d) or shifted to 32 °C (heat stress) (e). Survival of the animals was monitored. For detailed statistics see Supplementary Table4. Source data underlying Fig.6c–eare provided as a Source Data file. We propose that this function is the major reason why PP4 SMK-1 is required for the induction of many DAF-16 target genes under low IIS. The relevant substrate of PP4 SMK-1 is SPT-5 We now had identified the steps in the cascade from DAF-16 activation to target gene expression which depend on PP4 SMK-1 . But PP4 SMK-1 is a phosphatase, and we still did not know the relevant substrate whose dephosphorylation influences Pol II recruitment and behavior at a subset of DAF-16 target genes. First we took a candidate approach to test whether DAF-16 itself could be the target. However, neither our IP–MS/MS experiments (Fig. 1a, b , Supplementary Tables 2 , 3 , and ref. [17] ) nor published co-IPs [8] provided evidence for a physical interaction between PP4 SMK-1 and DAF-16. In addition, we investigated the smk-1 -dependent phosphorylation status of DAF-16 by phos-tag gel-electrophoresis. We grew DAF-16::GFP-expressing C. elegans containing either daf-2(e1370) or daf-18(mg198) and exposed them to either control or smk-1 by RNAi. As expected from high IIS activity leading to phosphorylation of DAF-16, we observed an upshift of DAF-16::GFP in daf-18 versus daf-2 mutant protein extracts when analyzed by a phos-tag gel and western blotting, but RNAi of smk-1 had no effect on the migratory behavior of DAF-16::GFP in this assay (Supplementary Fig. 7 ). All this data argued that the relevant substrate of PP4 SMK-1 is distinct from DAF-16. To identify the relevant substrate, we turned to an unbiased phosphoproteomics approach. We grew daf-2 mutant animals to scale, treated them with either control or smk-1 RNAi, lysed them, and determined their phosphoproteome by TiO 2 -based phosphopeptide enrichment and LC–MS/MS (see also Fig. 6a ). 208 phosphopeptides whose abundance increased upon smk-1 RNAi—and thus should be direct or indirect targets of PP4 SMK-1 —could be identified (Fig. 6a , Supplementary Table 7 ). The phosphopeptides originated from 150 proteins (Supplementary Table 7 ), of which we selected 41 for further evaluation based on their annotation and the significance of their smk-1 -dependent differential phosphorylation. 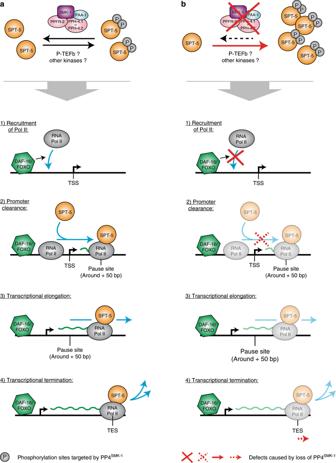Fig. 7: Model illustrating the roles of PP4SMK-1and SPT-5 for the transcription of DAF-16/FOXO target genes. SPT-5 is known to get phosphorylated at various sites. Some of these sites, in particular proline-directed sites in the SPT-5 CTD, are targeted by the kinase P-TEFb, to promote transcriptional elongation. However, our study shows that other phosphorylation events in- and outside the SPT-5 CTD occur, too. We do not know the kinases which phosphorylate these other sites, be it P-TEFb or rather distinct kinases. However, we found that several of these other sites are dephosphorylated by the phosphatase PP4SMK-1.aNormally, the phosphorylation state of these PP4SMK-1-targeted sites is in balance. We unfortunately do not know during which stages of transcription they are phosphorylated nor when their dephosphorylation by PP4SMK-1has to occur; but ultimately this balance allows for the efficient expression of DAF-16 target genes under low IIS.bIn contrast, when PP4SMK-1activity is missing, this balance shifts toward an overabundance of SPT-5 that is phosphorylated at these sites. Even though we do not understand the full mechanistic basis to it, this shift toward increased SPT-5 phosphorylation interferes with Pol II recruitment to promoter regions and may also mildly affect promoter clearance, leading to impaired transcription initiating events. Finally, a mild delay in transcriptional termination may occur, too. The red crosses and arrow indicate these phenotypes. To determine the functional relevance of these candidate proteins, we used a transcriptional reporter for the canonical DAF-16 target gene sod-3 . This reporter is induced by DAF-16 under low IIS—an induction that requires SMK-1 [8] . Hence we knocked down each of the 41 candidates by RNAi in wild type or daf-2 mutant animals carrying Psod-3::GFP and evaluated their GFP expression from day 1 to day 3 of adulthood. Knockdown of several candidates led to substantial changes in the expression of this reporter (Fig. 6b , Supplementary Fig. 8a ). We additionally searched our SMK-1 IP–MS/MS data to see whether any of these candidates co-purified with PP4 SMK-1 , a behavior that often can be observed for phosphatase substrates [25] . Indeed, we found that several of our candidate substrates co-purified with SMK-1 (Figs. 1b and 6b , Supplementary Tables 2 , 3 ). Together, these analyses highlighted one candidate in particular—the evolutionarily conserved protein SPT-5, which is predominantly known as a transcriptional elongation factor (Fig. 6b ). Firstly, SPT-5 influences the expression of sod-3 (Fig. 6b , Supplementary Fig. 8a ). Secondly, SPT-5 harbors four phosphorylation sites that become more phosphorylated in the absence of PP4 SMK-1 under low IIS (Fig. 6b , Supplementary Table 7 ). This differential phosphorylation of SPT-5 had the best p value of all sod-3 -influencing candidates. Thirdly, SPT-5 physically associated with PP4 SMK-1 according to our IP–MS/MS data (Figs. 1b and 6b , Supplementary Table 3 )—an interaction that we were able to validate even between the human orthologs of SMK-1 and SPT-5 in HEK293T cells (Supplementary Fig. 8c ). Finally, two additional transcription elongation factors from the same SPT family which closely synergize with SPT-5 [26] emerged from our study: (1) EMB-5 [27] , which just like SPT-5 is a candidate substrate of PP4 SMK-1 (Fig. 6b ); and (2) SPT-4, which just like SPT-5 can be bound by PP4 SMK-1 (Supplementary Table 3 ) and which together with SPT-5 forms the so-called DSIF (DRB sensitivity inducing factor) complex, involved in regulating Pol II’s promoter-proximal pausing and transcriptional elongation [28] . We then tested the consequences of losing any of these SPT family members for DAF-16-driven longevity and the increased resistance to oxidative and heat stress under low IIS. Already during the sod-3 reporter assays we observed that RNAi of spt-5 and emb-5 from the L1 stage leads to developmental arrest. This is not surprising, as they should be essential for transcription throughout the genome [24] . Hence we conducted knockdowns of spt-4 from the L1 or L4 stage, while spt-5 and emb-5 were knocked down from the L4 stage to overcome developmental phenotypes and hopefully leave behind sufficient residual amounts of these proteins to retain a basic level of genome-wide transcription. In these experiments, RNAi of emb-5 or spt-4 did not affect DAF-16-driven longevity under low IIS (Supplementary Fig. 8b ; L1 feeding data for spt-4 RNAi are not shown), leading us to exclude these SPT family members as relevant substrates. However strikingly, RNAi of spt-5 led to phenotypes perfectly reminiscent of smk-1 loss, namely impaired longevity and resistance to oxidative stress but not to heat stress in daf-2 mutant animals, while spt-5 RNAi had no effect in wild type or in daf-2; daf-16 animals (Fig. 6c–e ). Western blotting revealed that our knockdown eliminated ~92% of the SPT-5 protein (Supplementary Fig. 9a, b ), which indicated that as little as ~8% of the physiological amount of SPT-5 is sufficient to assure a basic level of genome-wide transcription but is insufficient to help PP4 SMK-1 promote the induction of DAF-16 target genes and therefore the mechanisms described in this study. Fig. 6: PP4 SMK-1 promotes DAF-16’s functions under low IIS by dephosphorylating SPT-5. Identification of the relevant PP4 SMK-1 substrate by unbiased phosphoproteomics and functional evaluation of the emerging candidates. a Workflow of the phosphoproteomics approach to identify PP4 SMK-1 substrate candidates, followed by their functional evaluation through RNAi screening using a sod-3P::GFP reporter in either wild type or daf-2(e1370ts) backgrounds. b Results from the approach shown under a . The table is limited to proteins that were found significantly more phosphorylated upon smk-1 RNAi and that additionally affected expression of sod-3 , i.e., by sod-3 induction in wild type or the repression of sod-3 expression in daf-2(e1370ts) mutant animals. The table is ranked by the significance ( p value) of the increased phosphorylation observed upon smk-1 RNAi. SPT-5 is highlighted in red as being the top-ranked candidate from this prioritization approach. c – e Loss of SPT-5 phenocopied the stress resistance and lifespan phenotypes caused by loss of SMK-1. All strains used in in this figure harbored the eri-1(mg366ts) mutation to yield better knockdown efficiencies [51] . Wild type, daf-2(e1370ts) , or daf-16(mgDf47lf) ; daf-2(e1370ts) mutant animals were grown from the L4 stage on either control or spt-5 RNAi bacteria at 25°C. Animals remained either untreated ( c ), or were grown until day 2 of adulthood and then transferred to either 6 mM tBOOH containing RNAi plates (oxidative stress) ( d ) or shifted to 32 °C (heat stress) ( e ). Survival of the animals was monitored. For detailed statistics see Supplementary Table 4 . Source data underlying Fig. 6c–e are provided as a Source Data file. Full size image Overall, this data is consistent with SPT-5 being a key substrate by which PP4 SMK-1 influences Pol II at many DAF-16 target genes and thereby fulfills its lifespan and stress resistance regulatory roles under low IIS. SPT-5 is a direct substrate of PP4 SMK-1 Having identified SPT-5, we wanted to test if it is a direct or rather an indirect substrate of PP4 SMK-1 . To address this, we conducted in vitro phosphatase assays. First, we immunoprecipitated the PP4 SMK-1 complex from C. elegans and transferred it to the appropriate assay buffer. Next, we incubated the complex with a variety of different synthetically made phosphopeptides which resembled the four PP4 SMK-1 -dependent phosphosites that we had identified by our phosphoproteomics. As a negative control, we incubated the complex with a phosphopeptide that is known to be targeted by the closely related phosphatase PP2A [29] . Remarkably, we found that PP4 SMK-1 selectively dephosphorylated two of these phosphosites in SPT-5, S677, and S882, while it did not dephosphorylate the other phosphosites nor the negative control peptide (Supplementary Fig. 9c ). To further confirm that this dephosphorylation was truly caused by PP4 SMK-1 and not other C. elegans proteins or contaminants that might co-purify with the complex, we expressed a minimal PP4 SMK-1 complex comprised of C. elegans PPH-4.1, PPFR-2, and SMK-1 recombinantly in S. cerevisiae . We purified this complex (see also Supplementary Fig. 9d ), transferred it to assay buffer and conducted the same in vitro phosphatase assay as previously. Similar to the PP4 SMK-1 complex purified from C. elegans , the recombinantly expressed minimal PP4 SMK-1 complex also selectively dephosphorylated the sites S677 and S882 (Supplementary Fig. 9e ). Finally, we tried to explore the purpose of the regulatory subunits, including SMK-1, in the PP4 SMK-1 complex. Other studies have shown that regulatory subunits of PP4 can confer substrate binding and specificity [10] , [11] , [30] , [31] . Thus, we repeated our in vitro phosphatase assay one more time, now using only the catalytic subunit of PP4 SMK-1 , PPH-4.1, which we recombinantly expressed in E. coli . Notably, even though PPH-4.1 was sufficient to dephosphorylate the PP4 SMK-1 -targeted sites in vitro, the enzyme had now lost its selectivity and also dephosphorylated the SPT-5 phosphosite S904 or the PP2A target peptide with equal or even better efficiency (Supplementary Fig. 9f ). We conclude that PP4 SMK-1 selectively dephosphorylates at least two phosphorylation sites in SPT-5 in vitro, which provides strong support for SPT-5 being a direct and specific substrate of PP4 SMK-1 also in vivo. The transcription factor DAF-16/FOXO is one of the most central and powerful aging regulators across metazoans, relaying many distress signals into compensatory, aging-preventive transcriptional responses. Nevertheless, it is not self-sufficient but depends on other proteins’ assistance. SMK-1, the first protein of this kind to be discovered [8] , is essential for DAF-16 to promote longevity and the resistance to many stresses under low IIS. This makes SMK-1 an important aging regulator in itself. Despite this prominence and the thorough genetic exploration of its functions [8] , it had remained unknown how SMK-1 is acting mechanistically. We could show that SMK-1 functions as part and through the catalytic activity of a specific Protein Phosphatase 4 complex, PP4 SMK-1 , and identified a direct substrate of this complex, SPT-5, whose dephosphorylation appears important for promoting DAF-16 functions under low IIS. But how does PP4 SMK-1 -driven dephosphorylation of SPT-5 promote target gene expression by DAF-16? The literature describes SPT-5 predominantly as a transcriptional elongation factor and part of the conserved DSIF complex which it forms together with SPT-4 [32] . This complex binds to Pol II during transcriptional initiation and remains associated with it throughout transcription [33] , [34] . DSIF is important for Pol II’s promoter-proximal pausing and transcriptional elongation [35] ; but specifically SPT-5 was found to influence also other stages of transcription. Under certain circumstances it can influence Pol II’s binding to promoter regions and transcriptional initiation [36] . This has been proposed to originate from elongation-engaged SPT-5 inferring epigenetic changes in promoter regions that facilitate new rounds of preinitiation complex (PIC) formation and thereby Pol II recruitment [36] . Furthermore, SPT-5 facilitates promoter clearance by outcompeting PIC components like TFIIE from association with Pol II [36] , [37] . And last but not least, SPT-5 can influence transcriptional termination [34] . Several of these functions depend on the phosphorylation status SPT5 [32] , [34] . Upon transcriptional initiation, Pol II and SPT-5 await elongation-promoting signals by the kinase P-TEFb, which usually phosphorylates both proteins at “proline-directed” sites (S/T-P) in their CTDs and thereby drives pause site release and transcriptional elongation [38] , [39] , [40] . SPT-5’s CTD remains phosphorylated throughout elongation and is dephosphorylated again near the transcriptional end site (TES), which contributes to transcriptional termination and release of Pol II and the DSIF complex from DNA [34] . In yeast, this dephosphorylation is conferred by Protein Phosphatase 1 (PP1) [34] . All this prior work has already shown that SPT-5, even though it is mostly known as an elongation factor, can in principle influence most stages of transcription and that the phosphorylation state of SPT-5 is important for these roles. Such is consistent with our study showing that dephosphorylation of SPT-5 by PP4 SMK-1 promotes transcription initiating events at DAF-16 target genes under low IIS. Only how this works exactly remains an open question. The actual phosphorylation status of the PP4 SMK-1 -targeted sites in SPT-5 during the different stages of transcription as well as off the DNA remains unknown. We can only say that they are overall hyperphosphorylated upon smk-1 RNAi and that none of these sites, even though some of them are located within SPT-5’s CTD, are the canonical P-TEFb target sites mentioned above. Thus, we also do not know if PP4 SMK-1 directly counteracts P-TEFb or whether it may dephosphorylate sites targeted by other kinases. The exact role of all phosphorylation sites on SPT-5 both inside and outside of its CTD, their turnover in the course of transcription, and the full portfolio of kinases and phosphatases that target them will be interesting topics of future investigation. We would like to note that PP4 SMK-1 predominantly promotes the step of Pol II recruitment to promoter regions, which is an event when SPT-5 has not yet bound to Pol II. Thus, in this context the effect of SPT-5 on Pol II should be indirect, which by analogy to previous observations [36] may be caused by elongation-engaged SPT-5 conferring epigenetic changes in promoter regions that facilitate Pol II recruitment. In a last effort to supplement our understanding of the PP4 SMK-1 –SPT-5–Pol II regulatory axis described in our study, we addressed three remaining questions. First, is it possible that PP4 SMK-1 impacts transcription initiating events by regulating SPT-5’s recruitment to promoter/TSS regions? We addressed this by ChIP-seq analysis of DAF-16/SMK-1 co-activated genes in daf-2 animals and found that knockdown of smk-1 had no significant effect on SPT-5 recruitment (Supplementary Fig. 10a ). This suggests that it is not absence of SPT-5 but its altered phosphorylation status that impairs transcription initiating events in the absence of PP4 SMK-1 . Second, we asked if, analogous to PP1 in yeast, PP4 SMK-1 also influences transcriptional termination. Again through ChIP-seq in daf-2 animals, we observed that smk-1 RNAi causes a moderate shift of SPT-5 and Pol II distribution into the downstream direction, specifically at TESs of DAF-16/SMK-1-co-activated genes (Supplementary Fig. 10b, c ). This result would be consistent with also transcriptional termination being moderately delayed at these genes. However, it remains to be tested whether and to what extend such termination defects would actually contribute to reduced expression of these genes. Third, we asked where PP4 SMK-1 encounters SPT-5 and dephosphorylates it. We conducted ChIP-seq of SMK-1 using SMK-1::GFP-expressing daf-2 mutant C. elegans . Association of SMK-1 with chromatin was extremely weak. However when looking cumulatively at all genes genome-wide, we observed a profile that would be consistent with SMK-1 binding to SPT-5 specifically during transcriptional elongation and dissociating just before the TES is reached (Supplementary Fig. 10d ). This data argues that dephosphorylation of SPT-5 by PP4 SMK-1 may occur during transcriptional elongation prior to termination. However, we cannot exclude that PP4 SMK-1 acts also in the nucleoplasm, where it would dephosphorylate SPT-5 to prepare it for engagement in new rounds of transcription. A remarkable aspect of our study is that PP4 SMK-1 influences transcription through a highly conserved and common component of the transcription regulatory machinery, namely SPT-5. Nevertheless, it does not affect transcription genome-wide but only of a limited gene set. Such specificity actually has precedence. Studies in zebrafish and flies have similarly shown that mutations of SPT-5 affect only parts of the transcriptome [41] , [42] . But where would this specificity come from? We could see in Fig. 5c that promoter regions of DAF-16/SMK-1-co-activated genes may have unique properties, resulting in Pol II clearing these promoter regions more slowly. We propose that this makes them more sensitive to defects in transcription initiating events. Looking for sequence features that may distinguish these promoter regions, we found them enriched for TATA-boxes (TATA) ( p = 2.45 × 10 −4 ; Supplementary Table 8 ), while initiator elements (Inr) were not enriched (Supplementary Table 8 ). In contrast, DAF-16-activated promoters that do not depend on SMK-1 for their activation are depleted of both TATA and Inr (Supplementary Table 8 ). Notably, presence of TATA-boxes has been associated with genes for which transcriptional initiation is particularly rate limiting [43] . Considering all these observations, it would be consistent that loss of PP4 SMK-1 and the resulting impairment of transcription initiating events selectively impair the expression of this subset of DAF-16 target genes. Regarding the purpose of such regulatory mechanism we can only speculate. It may be a feature of genes that need the ability to be rapidly and/or robustly induced in response to certain stimuli, i.e., a drop in IIS. Consistent with such notion, a recent study in humans showed particular involvement of SPT-5 in regulating the transcriptional initiation of rapidly-induced immune response genes [36] . Nevertheless, future studies will have to explore this in more detail. It is also notable that PP4 SMK-1 , although it is required for most DAF-16 functions under low IIS, is irrelevant for some, e.g., for promoting resistance to heat stress (Fig. 3 ). Consistently, we observed that depletion of SPT-5 impaired longevity and oxidative stress resistance but not heat stress resistance under low IIS (Fig. 6c–e ). This indicates that some DAF-16 target genes are regulated in a fundamentally different manner that does not involve the PP4 SMK-1 –SPT-5–Pol II axis, e.g., due to different promoter characteristics or DAF-16 fulfilling these functions in synergy with other transcription factors that impose different mechanisms of transcriptional control at these loci. Intriguingly, for heat shock response genes it is already known that DAF-16 regulates them combinatorially together with HSF-1 [44] ; and it has been shown that expression of HSF-1 target genes is not controlled on the level of Pol II recruitment or promoter clearance but rather by pause site release [45] . Taken together, our study provides substantial mechanistic insight and suggests a possible model for how SMK-1 promotes the expression of many DAF-16-activated genes under low IIS. Figure 7 illustrates this model and highlights the transcriptional events that seem affected when PP4 SMK-1 activity is missing. Fig. 7: Model illustrating the roles of PP4 SMK-1 and SPT-5 for the transcription of DAF-16/FOXO target genes. SPT-5 is known to get phosphorylated at various sites. Some of these sites, in particular proline-directed sites in the SPT-5 CTD, are targeted by the kinase P-TEFb, to promote transcriptional elongation. However, our study shows that other phosphorylation events in- and outside the SPT-5 CTD occur, too. We do not know the kinases which phosphorylate these other sites, be it P-TEFb or rather distinct kinases. However, we found that several of these other sites are dephosphorylated by the phosphatase PP4 SMK-1 . a Normally, the phosphorylation state of these PP4 SMK-1 -targeted sites is in balance. We unfortunately do not know during which stages of transcription they are phosphorylated nor when their dephosphorylation by PP4 SMK-1 has to occur; but ultimately this balance allows for the efficient expression of DAF-16 target genes under low IIS. b In contrast, when PP4 SMK-1 activity is missing, this balance shifts toward an overabundance of SPT-5 that is phosphorylated at these sites. Even though we do not understand the full mechanistic basis to it, this shift toward increased SPT-5 phosphorylation interferes with Pol II recruitment to promoter regions and may also mildly affect promoter clearance, leading to impaired transcription initiating events. Finally, a mild delay in transcriptional termination may occur, too. The red crosses and arrow indicate these phenotypes. Full size image Intriguingly, SMK-1 may influence not only the expression of DAF-16-dependent genes but also the targets of other transcription factors, and it may promote longevity also in conditions besides low IIS. We obtained preliminary support for this notion when we compared the genes regulated by SMK-1 under low IIS to the genes regulated by two other transcription factors that also contribute to the longevity of daf-2 mutant C. elegans —SKN-1 [46] and HLH-30 [18] . In particular, genes regulated by HLH-30 were strongly dependent on SMK-1 for their regulation (Supplementary Table 9 ). A previous study investigating dietarily restricted C. elegans ( eat-2 mutants) showed that their longevity, which depends not on DAF-16 but rather PHA-4, was also dependent on SMK-1 [47] . Finally, it was shown that SMK-1 is essential for the increased lifespan of mitochondrial electron transport chain mutants [8] . This points to an involvement of PP4 SMK-1 also with other aging-regulatory signaling pathways and their downstream transcription factors, which will be interesting to explore further. 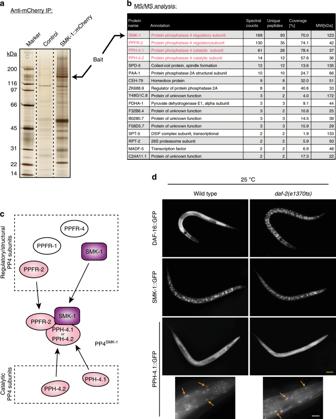Finally we would like to highlight the strong conservation of all components mentioned in our study across metazoans. Two previous studies in S. cerevisae have observed a physical interaction between Psy2 (the S. cerevisiae ortholog of SMK-1) and Spt5 in tandem affinity purification-MS/MS experiments [9] , and we were able to confirm the existence of a PP4 SMEK -SUPT5H complex under low IIS conditions in human cells (Supplementary Fig. 8c ). This suggests that a PP4 SMEK –SUPT5H–Pol II axis influencing the expression of FOXO target genes might exist in humans, too. It will be important to verify its conservation and whether it likewise promotes stress resistance and longevity. Fig. 1: SMK-1 is part of a globally expressed nuclear Protein Phosphatase 4 complex. aSDS-PAGE and silver staining analysis of an anti-mCherry immunoprecipitation from whole-animal lysates ofC. elegansexpressing SMK-1::mCherry. Animals expressing no transgene were used as negative control.bList of the proteins identified in the purification froma, as determined by mass spectrometry (LC–MS/MS). Only proteins identified by at least two unique peptides are shown. See also Supplementary Table2for an independent repeat of this experiment.cModel illustrating the composition of the specific Protein Phosphatase 4 complex (PP4SMK-1) that co-purified with SMK-1, next to other implicated PP4 subunits not found in this complex.dLocalization studies of DAF-16::GFP, SMK-1::GFP, and PPH-4.1::GFP in wild type and indaf-2(e1370ts)mutant animals. Worms were grown from the L1 stage at 15 °C, then shifted to 25 °C at the L2/L3 stage. After 16 h the GFP signal was recorded in L4 animals (yellow scale bar: 100 µm). The higher magnification images for PPH-4.1::GFP show head regions. Arrows are highlighting the partial nuclear accumulation of PPH-4.1 in both wild type anddaf-2(e1370ts)animals (white scale bar: 20 µm). C. elegans strains and alleles For a complete list of strains used in this study, see Supplementary Table 1 . Alleles obtained from other labs were 4 times outcrossed to the lab’s N2 background. All C. elegans strains were grown and maintained on Escherichia coli OP50 using standard methods [48] . RNAi by feeding C. elegans were grown on the E. coli strain HT115 containing dsRNA-expressing plasmids targeting the genes of interest. RNAi clones either were obtained from published collections [49] , [50] or were newly made. RNAi clones for daf-2 , pph-4.1, pph-4.2, ppfr-2, spt-4 , and emb-5 were used from [49] and RNAi clones for daf-16 , spt-5 , and smk-1 were used from [50] . For screening purposes, all available RNAi clones from [49] , [50] that targeted the genes of interest were used. RNAi clones targeting ppfr-1 and ppfr-4 were newly made by PCR-amplifying approximately 1 kb of cDNA or gDNA sequence located in the coding region of the gene of interest, cloning it into L4440 by AT-ligation, and then transforming the resulting construct into E. coli HT115. PCR primers CAACAACTTGGCGGTGCTATC (forward) and GTTCCGGATTGCAAGCAACG (reverse) were used on gDNA to make the ppfr-1 RNAi clone; and CAAGCGCTTTACGATCCGAG (forward) and CATCCACGTCGATGATCATCC (reverse) were used on cDNA to make the ppfr-4 RNAi clone. E. coli HT115 containing the empty plasmid L4440 served as negative control in the RNAi experiments. Combined knockdown of either the two PP4 SMK-1 catalytic subunits pph-4-1 and pph-4.2 or of pph-4.2 and smk-1 was achieved by a 1:1 mixture of their RNAi bacteria. Unless stated otherwise, RNAi feeding was initiated at the L1 stage. In most RNAi experiments, a RNAi-sensitized strain background ( eri-1(mg366) ) was used, to yield better knockdown efficiency [51] . Usage of this background is always stated in the respective figure legends. Generating transgenic C. elegans To generate PPH-4.1::GFP-expressing C. elegans , the promoter of pph-4.1 (the first 600 bp upstream of the START codon) was cloned from genomic DNA and the spliced pph-4.1 coding region from cDNA of N2 animals. These sequences were then fused by PCR and cloned into the GFP-fusion expression vector pPD95_75 (Addgene), to yield the desired pph-4.1P::pph-4.1::gfp construct. Next, we coinjected this plasmid (30 ng/µl) with ScaI-digested pUC19 (40 ng/µl) and EcoRI-digested pRF4 (30 ng/µl) to yield complex arrays marked by rol-6(su1006) . Injections were performed using an inverted DIC microscope (Zeiss) in combination with an InjectMan 4 and FemtoJet 4i (Eppendorf). Rollers were selected from the F1 progeny and lines were established. C. elegans expressing catalytically dead PPH-4.1(R262L) were generated in the same way—only that we mutated the pph-4.1P::pph-4.1::gfp construct by site-directed mutagenesis, replacing AGA by CTT. Microscopy and nuclear translocation assays For imaging, L4 stage worms were paralyzed by 2,3-butanedione monoxime (BDM), mounted on 2% agarose pads, and imaged using a Zeiss Axio Observer Z1 microscope at 20x or 40x magnifications. To investigate the effect of SMK-1 on nuclear entry of DAF-16, daf-2(e1370) mutant animals expressing DAF-16::GFP were grown from the L1 stage at 15 °C on either control or smk-1 RNAi. On day 2 of adulthood, animals were shifted to 25 °C, upon which moment nuclear entry was scored in the intestine of the animals. To investigate the effect of SMK-1 on nuclear exit of DAF-16, animals were grown in the same way to day 1 adulthood, shifted to 25 °C for 24 h to reach full nuclear entry of DAF-16, and then shifted back to 15 °C, upon which moment nuclear exit was scored in the intestine of the animals. Scoring was done blinded, using a Zeiss Axio Zoom V16 microscope. Testing the knockdown efficiency of spt-5 RNAi daf-2(e1370) animals expressing SPT-5::GFP were synchronized by bleaching, grown on HT115 bacteria without dsRNA-expressing plasmids at 15 °C until the L4 stage, washed in antibiotics to remove the HT115, and transferred to plates seeded with either control or spt-5 RNAi bacteria. 5-fluoro-2′-deoxyuridine (FUDR) was added to a final concentration of 50 µM to prevent progeny production and the plates were shifted to 25 °C. On day 2 of adulthood, 50 worms per condition were harvested and analyzed by SDS-PAGE and western blotting. For detection of SPT-5::GFP we used monoclonal mouse anti-GFP antibody (Roche) and for detection of actin we used monoclonal (C4) mouse anti-actin antibody—both diluted 1:1000 in TBST containing 5% milk powder. For quantification, band intensities were determined using the Fiji image processing package (ImageJ) and data were normalized to actin. This experiment was repeated 3 times. Unpaired t test (two-tailed) was used for comparisons and statistical analysis. Lifespan assays C. elegans were synchronized by bleaching and grown, depending on the experiment, on either OP50 or RNAi bacteria at 15 °C until the late L4 stage. In cases where the RNAi bacteria would lead to developmental arrest, animals were initially grown on HT115 bacteria without dsRNA-expressing plasmids at 15 °C and only at the L4 stage washed in antibiotics to remove the HT115 and transferred to RNAi bacteria. In all cases 5-fluoro-2′-deoxyuridine (FUDR) was added to a final concentration of 50 µM at the late L4 stage to prevent progeny production and the plates were shifted to 25 °C. Survival of animals was determined every 2–3 days by scoring movement upon prodding with a platinum wire [52] . Stress survival assays C. elegans were synchronized by bleaching and grown, depending on the experiment, on either OP50 or RNAi bacteria at 15 °C until the late L4 stage. In cases where the RNAi bacteria would lead to developmental arrest, animals were initially grown on HT115 bacteria without dsRNA-expressing plasmids at 15 °C and only at the L4 stage washed in antibiotics to remove the HT115 and transferred to RNAi bacteria. In all cases FUDR (50 µM final concentration) was added at the late L4 stage to prevent progeny production and the plates were shifted to 25 °C. At day 2 of adulthood, animals were transferred to plates containing 6 mM tBOOH (for oxidative stress assays), the temperature was shifted to 32 °C (for heat stress assays), or animals were exposed to 1500 J/m 2 UV light (for UV stress assays). Their survival was recorded and analyzed by a fully automated lifespan machine [16] . Immunoprecipitation from C. elegans Growth of C. elegans to large scale, harvesting, lysis, IP of the bait proteins, and eventual analysis of the precipitated material by tandem mass spectrometry were conducted as previously described [17] . At first, the animals were grown asynchronously at 15 °C to scale, then shifted for 16 h to 25 °C and harvested. Animals were transferred to lysis buffer (50 mM HEPES at pH 7.4, 1 mM EGTA, 1 mM MgCl2, 150 mM KCl, 10% (v/v) glycerol, Complete without EDTA (Roche), 1 mM phenylmethyl sulphonyl fluoride, and phosphatase inhibitors (Sigma)) and lysed by grinding under liquid nitrogen. NP-40 was added to 0.05% (v/v), and the resulting lysate was cleared at 20,000 g. mCherry-tagged bait proteins were immunoprecipitated using a rabbit-anti-mCherry antibody that we generated in the lab and coupled to Protein A resin (Biorad). GFP-tagged bait proteins were immunoprecipitated using GFP-trap resin (Chromotek). Immunoprecipitated proteins were eluted using 100 mM glycine at pH 2.6. As negative controls for background subtraction, the same purifications and later mass spectrometry analyses were conducted using wild type (untagged) C. elegans . Mass spectrometry to identify co-purifying proteins Immunoprecipitated proteins were digested overnight at pH 8.3 using sequencing-grade trypsin. Resulting peptides were separated by microcapillary reverse-phase chromatography and identified by online tandem mass spectrometry using an LTQ Orbitrap XL hybrid linear ion trap-orbitrap high-resolution mass spectrometer (Thermo). Tandem mass spectra produced by collision induced dissociation (CID) in the ion trap were searched against the Wormpep database (version 246) using ProLuCID [53] and DTASelect [54] . Enzyme specificity was set to trypsin, allowing cleavage N-terminally to proline. Further modifications were cysteine carbamidomethylation (fixed), as well as methionine oxidation and phosphorylation of the amino acids S,T, or Y (all variable). False discovery rates (FDRs) were determined by searching the mass spectra against the reversed sequences of the Wormpep database. Proteins had to be identified by at least two independent peptides, resulting in an FDR below 1%. Finally, samples were compared using Contrast [54] . Any proteins that were identified also in the control purifications (from untagged C. elegans lysates) were likely contaminants and thus eliminated from Fig. 1b and Supplementary Tables 2 , 3 . Co-immunoprecipitation from HEK293T cells The HEK293T cells (ATCC, tested to be void of mycoplasma contamination) were grown in advanced Dulbecco’s modified Eagle’s medium/F12 supplemented with 10% fetal bovine serum and then transfected in 9 cm dishes with 15 μg of plasmid DNA for GFP-SMEK1 (Addgene), using the Profection mammalian transfection system (Promega). 12 h post transfection, medium was replaced with fresh antibiotic-free media and LY294002 was added at a final concentration of 20 μM. After 48 h of LY294002 treatment, cells were harvested by scraping and frozen in liquid nitrogen. For the co-IPs, these cell pellets were thawed into lysis buffer (50 mM HEPES at pH 7.4, 1 mM EGTA, 1 mM MgCl2, 150 mM KCl, 10% (v/v) glycerol, Complete (Roche), 1 mM phenylmethyl sulphonyl fluoride, phosphatase inhibitors (Roche), and 0.5% (v/v) NP-40) and lysed by shearing through a G30 syringe. Lysates were cleared at 20,000 g. GFP-tagged proteins were immunoprecipitated using GFP-Trap resin (Chromotek) and eluted by boiling in 2× sample buffer. Input (IN) and eluate (IP) samples were analyzed by SDS-PAGE and western blotting. Production of recombinant proteins in E. coli The cDNA of pph-4.1 was cloned into the GST-fusion expression vector pGEX-4T1 and the resulting plasmid transformed into BL21(DE3)-RIPL (Agilent). The resulting bacterial strain was grown to an OD 600 of 0.6 at 37 °C and 230 rpm and then induced with IPTG for 18 h at 18 °C and 230 rpm. Next the bacteria were harvested and frozen in liquid nitrogen. For the purification of PPH-4.1, the bacteria were thawed into TBS buffer containing 1 mM EDTA, 1 mM DTT, and Complete without EDTA (Roche), and incubated with lysozyme for 30 min at 4 °C. Resulting lysate was sonicated, Triton X-100, RNase A (Roche), and DNase I (Invitrogen) were added to concentrations of 1% (v/v), 10 µg ml −1 , and 5 µg ml −1 , respectively, and the lysate then incubated for another 30 min at 4 °C. Glutathione-Sepharose 4B resin (GE Healthcare) was added to the lysate and incubated rotating for 2 h at 4 °C. Finally, the resin was washed in TBS, resuspended in TBS, and then used for in vitro phosphatase assays. Production of recombinant proteins in S. cerevisiae The cDNA of pph-4.1 was fused to a TAP tag and then used to replace the cdt1 gene in the plasmid pJF2 [55] , creating a Gal1 promoter-driven expression construct. The cDNA of ppfr-2 was used to replace mcm7 and the cDNA of smk-1 was fused to a HA 3 tag and then used to replace mcm6 in the plasmid pJF4 [55] , creating a Gal1-10 promoter-driven expression construct. Both expression constructs were integrated into the genome of the S. cerevisiae strain CB3245 (MATa, pep4∆::HPH). Resulting cells were grown at 30 °C and 200 rpm in YEP medium containing 2% raffinose to an OD 600 of 1.0, then 2% galactose was added to induce the overexpression and the cells were grown for an additional 4 h at 30 °C and 200 rpm. Cells were harvested by centrifugation, washed with IPP150 buffer (50 mM Tris-HCl (pH 8.0), 150 mM NaCl, 10% glycerol, 0.1% NP-40, and 1 mM dithiothreitol (DTT)) and ground in liquid nitrogen using a SPEX 6870 freezer mill. Ground cells were dissolved in 1 ml IPP150 buffer containing Complete without EDTA (Roche), 10 mM MgCl 2 and 12.5 U Benzonase (Sigma), and incubated for 1 h at 4 °C. The lysate was cleared by centrifugation for 20 min at 16.000 g , and the purification of the TAP-tagged protein was performed as described before [56] with slight modifications. As beads for the purification we used IgG Sepharose 6 Fast Flow (GE Healthcare). Glutathione-Sepharose 4B beads (GE Healthcare) were used for the mock purification. Beads were divided into two tubes and washed with GF150 buffer (20 mM HEPES (pH 7.5), 150 mM NaCl, 10% glycerol, 0.1% NP-40, and 1 mM DTT). Finally, the PPH-4.1::TAP was eluted with TEV protease and used for in vitro phosphatase assays. For detection of PPH-4.1::TAP by western blotting we used anti-TAP antibody (antibodies online.com, Cat#ABIN398491) diluted 1:1000 in TBST containing 2% (w/v) milk powder (Sigma). For detection of SMK-1::HA 3 , we used anti-HA antibody (Abcam, cat # ab9110) diluted 1:3000 in TBST containing 5% (w/v) milk powder. PP4 SMK-1 purification from C. elegans for in vitro assays daf-2(e1370) animals expressing SMK-1::GFP were grown asynchronously to scale at 15 °C, then shifted for 16 h to 25 °C and harvested. Animals were transferred to lysis buffer (50 mM HEPES at pH 7.4, 1 mM EGTA, 1 mM MgCl 2 , 150 mM KCl, 10% (v/v) glycerol, Complete without EDTA (Roche)), and lysed by grinding under liquid nitrogen. NP-40 was added to 0.05% (v/v), and the resulting lysate was cleared at 20,000 g. The SMK-1::GFP was immunoprecipitated using GFP-trap resin (Chromotek), the resin washed, and then resuspended in IP-EL buffer (50 mM HEPES at pH 7.4, 1 mM EGTA, 1 mM MgCl 2 , 150 mM KCl, and 10% (v/v) glycerol), to be used in the in vitro phosphatase assays. In vitro phosphatase assay We designed phosphopeptides for each PP4 SMK-1 -dependent phosphosite on SPT-5 (S671: PMVSRMAS(p)PNPMAS, S677: ASPNPMAS(p)PRHSSGG, S882: TPAYGS(p)ADGAR, S904: TPAYGS(p)TEGGR). In addition, we included a known PP2A substrate peptide (“PP2A target”), derived from the retinoblastoma protein RB [29] (PP2A target: INGSPRT(p)PRRGQNR), as a negative control. These peptides were synthesized (95% purity, TAG Copenhagen A/S) and, prior to assays, freshly diluted to 1 mM final concentration in pNPP Ser/Thr Assay Buffer (50 mM Tris-HCl (pH 7.0), 100 µM CaCl 2 ). Purified material (either 10 µl beads or 10 µl eluted protein) was mixed with 40 µl of 1 mM Phosphopeptide solution. Samples were incubated at RT for 15 min on a shaking incubator at 800 rpm. All these assays were conducted in triplicate. For the eventual detection of the released phosphate, samples were transferred to 96-well half area assay plates (Corning) and diluted fivefold in pNPP Ser/Thr Assay Buffer to reach detectable range. We used a Malachite Green Phosphate Assay Kit (Sigma, cat # MAK307) and performed the assay according to the manufacturer’s instructions. One-way ANOVA and post hoc Dunnett’s test were used for statistical calculations and multiple comparisons of each sample with the control substrate (“PP2A target”). Phos-tag SDS-PAGE analysis Worms were grown on either control or smk-1 RNAi bacteria until day 2 of adulthood and then harvested into a lysis buffer (20 mM MOPS (pH 7.2), 15 mM MgCl 2 , 100 mM NaCl, 1% (v/v) Triton X-100, 1 mM DTT, Complete without EDTA (Roche), 1 mM phenylmethyl sulphonyl fluoride, and PhosSTOP (Roche)). Samples were lysed using a FastPrep and silicon carbide beads with 1.0 mm diameter (BioSpec). Per condition, material equivalent to 50 worms was loaded onto SuperSep Phos-tag (50 µM) 10% precast gels (Wako) and then analyzed by SDS-PAGE and western blotting. Monoclonal mouse anti-GFP antibody (Roche) diluted 1:1000 in TBST containing 5% milk powder was used to detect DAF-16::GFP in the different samples. Sample preparation for phosphoproteomic analyses daf-2(e1370) mutant worms were synchronized by bleaching, seeded as L1 larvae onto plates containing either control or smk-1 RNAi bacteria, and grown at 15 °C until the L4 stage. Plates were then shifted to 25 °C and FUDR (50 µM final concentration) was added to prevent progeny production. On day 2 of adulthood, animals were harvested, washed, and frozen in liquid nitrogen. Animals were lysed by grinding under liquid nitrogen, using a cryomill (Retsch). Then 300 mg of worm powder were thawed and 200 µl of the resulting lysate transferred to a new tube, where it was diluted with 300 µl of lysis buffer (8 M Urea, 1% SDS, 50 mM Tris pH 8.5, protease inhibitors (Roche), and phosphatase inhibitors (Roche)). Samples were then sonicated on ice to shear the DNA and cleared by centrifugation for 10 min at 4 °C and 20,000 g . Supernatants were transferred to new tubes and their protein concentration measured using BCA assay (Pierce). Six hundred micrograms of proteins were reduced by adding DTT to a final concentration of 5 mM and incubating for 1 h at 25 °C. Samples were then alkylated by adding iodoacetamide to a final concentration of 15 mM and incubating for 30 min in the dark at room temperature. Excess iodoacetamide was quenched by adding DTT to an additional 10 mM of final concentration. Proteins were isolated by methanol/chloroform precipitation, redissolved in 100 µl of 50 mM Tris pH 8.5 containing 8 M urea, and then diluted with an equal volume of 50 mM Tris pH 8.5. Proteins were digested by adding 10 µg of LysC (Promega) and incubating for 6 h at 24 °C and 300 rpm. Next, three volumes of 50 mM Tris pH 8.5 were added to reach a final urea concentration of 1 M. 10 µg of LC grade trypsin (Promega) was added and samples were incubated overnight at room temperature. After digestion, TFA was added to 0.5% (v/v) and samples were centrifuged for 10 min at 4 °C and 20,000 g. The pellet was discarded and the supernatant desalted using C18 SepPak cartridges (Waters). Phosphopeptides were enriched using a TiO 2 Phosphopeptide Enrichment and Clean-up Kit (Pierce) according to the manufacturer’s recommendations. Mass spectrometry for phosphoproteomic analyses Peptides were separated using a 50 cm EASY-Spray™ LC column (Thermo Scientific) and the EASY-LC 1000 chromatography system (Thermo Scientific). Separation was achieved by a 120 min linear gradient from 2 to 26% acetonitrile in 0.1% formic acid at a flow rate of 300 nL/min. Eluting peptides were ionized by electron spray and analyzed by an Orbitrap Fusion mass spectrometer (Thermo Fisher Scientific). The survey MS spectrum was acquired at a resolution of R = 120,000 in the range of m/z 200–2000. MS/MS data for the 20 most intense precursors were obtained using higher-energy collisional dissociation for ions with a charge z > 1 at a resolution of R = 15,000. Data analysis for phosphoproteomic analyses RAW data from the mass spectrometer were analyzed using MaxQuant 1.5.3.30 [57] . A FDR of 0.01 for proteins and peptides and a minimum peptide length of six amino acids were required. The Andromeda search engine [58] was used to search the MS/MS spectra against the Uniprot C. elegans database (WBcel235) combined with 262 common contaminants and concatenated with the reversed versions of all sequences. Enzyme specificity was set to trypsin, allowing cleavage N-terminally to proline. Further modifications were cysteine carbamidomethylation (fixed), as well as protein N-terminal acetylation, asparagine and glutamine deamidation, methionine oxidation, and phosphorylation of the amino acids S,T, or Y (all variable). Further evaluation of the data provided by MaxQuant was performed using R [59] . Proteins’ relative intensities were normalized to the total protein signal. Differences in relative protein abundances between treated and control samples were assessed by moderated t test using the R-package limma [60] . Benjamini–Hochberg correction for multiple comparisons was used. Transcriptional reporter assays The sod-3p::GFP -expressing C. elegans strains CF1553 or AS23 were synchronized by bleaching and seeded as L1 larvae onto plates containing RNAi bacteria, grown at 15 °C until the L4 stage, and then shifted to 25 °C. For each gene of interest, all RNAi clones available in the two major genome-wide collections [49] , [50] were tested and we then used the ones with the strongest phenotypes. Any RNAi clones that would lead to developmental arrests were retested by initially growing the animals on HT115 bacteria without dsRNA-expressing plasmids at 15 °C and only at the L4 stage washing them in antibiotics to remove the HT115 and transferring them to the respective RNAi bacteria and to 25 °C. In all cases, production of progeny was prevented by addition of FUDR (50 µM final concentration) at the late L4 stage. GFP expression was evaluated/scored by visual inspection from day 1 to day 3 of adulthood, using a Zeiss Axio Zoom V16 microscope. mRNA isolation and sequencing Worms were synchronized by bleaching and about 150 of them grown from the L1 stage at 15 °C on control, smk-1 , or daf-16 RNAi bacteria. At the L4 stage, the plates were shifted to 25 °C and FUDR (50 µM final concentration) was added to prevent production of progeny. 16 h later, 100 animals were collected, washed, and immediately frozen in liquid nitrogen. Total RNA was extracted using Trizol (Sigma). RNA quality was assessed by determining its RNA integrity number (RIN). We required all samples to have a RIN above 9. mRNA-seq libraries were constructed using a TruSeq RNA SamplePrep V2 kit (Illumina) according to the manufacturer’s instructions. Chromatin immunoprecipitation Approximately 800,000 C. elegans were used per condition in each experiment. Worms were either grown asynchronously at 15 °C on large plates seeded with OP50 bacteria or they were synchronized by bleaching, L1 larvae seeded onto plates containing either control or smk-1 RNAi bacteria, and the animals grown at 15 °C until the late L4 stage. For the RNAi experiments, FUDR (50 µM final concentration) was added to prevent production of progeny. The animals were then shifted to 25 °C, grown for another 16–18 h, harvested, and subjected to chromatin immunoprecipitation (ChIP) [17] . Briefly, ground frozen worm powder was crosslinked using 1% formaldehyde in PBS and sonicated. IP was performed using Protein A Dynabeads (Invitrogen) and either rabbit polyclonal anti-GFP antibody (Takara, Cat# 632592), mouse monoclonal anti-RNA Polymerase II antibody [8WG16] (BioLegend, Cat# 920102), or mouse monoclonal anti-RNA polymerase II antibody that specifically detects CTD repeats phosphorylated at Ser5 [4H8] (Abcam, Cat# ab5408). Protein–DNA complexes were then eluted from protein A beads, treated with RNase A and proteinase K, and the resulting DNA purified. Sequencing libraries of inputs and immunoprecipitated samples were constructed using a protocol optimized for small DNA quantities [61] . High-throughput sequencing For both multiplexed mRNA-seq and ChIP-seq libraries, single-end sequencing was conducted for 50 cycles on Illumina HiSeq 2000 sequencers according to the manufacturer’s instructions. Image analysis, base calling, and quality scoring were carried out in real time with the standard Illumina analysis pipeline using a phiX control. Processing of mRNA-seq reads and downstream analysis Reads were mapped to the C. elegans genome using TopHat (v2.0.8b) [62] and known gene model annotations (WS220), as well as the following parameters: --library-type fr-unstranded --b2-very-sensitive --min-coverage-intron 10 --min-segment-intron 10 --microexon-search --no-novel-juncs. Transcript abundance (FPKM, fragments per kilo base of transcript per million fragments) and differential expression was calculated using Cuffdiff (v2.1.1) from the Cufflinks software package [63] and the following parameters: -u --FDR 0.05 --upper-quartile-norm --compatible-hits-norm --library-type fr-unstranded. All conditions were analyzed at least by using two biological replicates. Replicates were mapped individually and then combined by Cuffdiff. All analyses were limited to protein-coding genes. Statistically significant differentially expressed genes (DEGs, in other words “up- and downregulated” genes), were identified by Cuffdiff, using a 5% FDR. 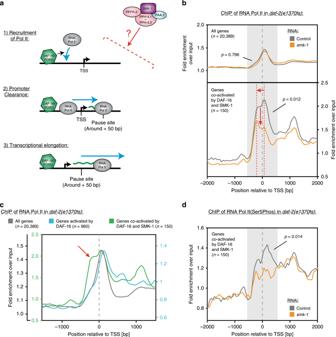Differential gene expression values were calculated as the ratio of FPKM values. To test for significant overlap between gene lists, we used the hypergeometric test (R function phyper [59] ). Fig. 5: PP4SMK-1is required for transcription initiating events at the genes co-activated by DAF-16 and SMK-1. aSchematic of the key steps that lead from DAF-16’s binding to promoter regions to the eventual transcription of the downstream genes.b–dChIP-seq analysis of RNA Pol II under low IIS.daf-2(e1370ts)mutant animals were synchronized and grown from the L1 stage on either control orsmk-1RNAi bacteria. At the L4 stage, animals were shifted to 25 °C. After an additional 16 h, animals were harvested and ChIP-seq analysis was conducted, using antibodies recognizing RNA Pol II, either in any modification state (b,c) or specifically RNA Pol II that was phosphorylated at Ser5 of its CTD (d). Average read densities across TSS regions of the indicated gene sets are shown.pvalues indicate the significance of read density differences in the grayed regions (−600 to +600 around the TSSs) between control andsmk-1RNAi treated animals. Source data underlying Fig.5b, d are provided as a Source Data file. Processing of ChIP-seq reads and metagene analysis For basic quality metrics of our ChIP-seq samples see Supplementary Table 5 . We aligned the reads to the C. elegans genome (WS220) by using Bowtie (v2.1) [64] with the following parameter: -q. Uniquely mapping reads that contained no more than one mismatch were used for peak calling and read density calculations. For the calculation of normalized read densities around TSSs, around transcriptional end sites (TESs; the sites where the transcribed region of the mRNA ends and polyadenylation begins), and at DAF-16 peaks, the R package ngs.plot [65] was used with the following parameters: -R tss -FL 200 (for TSSs), -R gene body -FL 200 (for TESs), or -R bed -E {bed-file of DAF16 peaks} -FL 200 (for DAF-16 peaks). The list of DAF-16 peaks was obtained from [17] . Using this software, read densities were calculated independently for input and IP samples in bins of 60 bp (Fig. 5b–d , Supplementary Figs. 4 d and 10a and for the regions outside the gene body in Supplementary Fig. 10b–d ) or of 1% of the gene body length (Supplementary Fig. 10b–d ). To then obtain the “fold enrichment over input” values which we plot in the figures, we divide the normalized IP read density of every bin by its corresponding input read density. For p value calculations determining whether DAF-16 binding to DAF-16 peak regions had significantly changed between the compared conditions, we first calculated the “fold enrichment over input” values in 60 bp bins, as stated above, covering a region from −600 to +600 bp around DAF-16 peak summits. Next, we compared the “fold enrichment over input” values in these bins between conditions using a t test [66] . p value calculations determining whether RNA Pol II, RNA Pol II(Ser5Phos), or SPT-5 binding to TSS regions had significantly changed between the compared conditions were conducted in identical manner, only that regions from −600 to +600 bp around TSSs were investigated. To calculate pausing indices from RNA Pol II ChIP-seq data, we first created an input-normalized BigWig file of IP data, using DeepTools [67] (function BamCompare with the following arguments: extendReads 200, operation ratio, binSize 60, scaleFactorsMethod None, normalizeUsing RPKM). For each gene, mean read coverages were calculated in specific regions (“relaxed” pausing region [−500 to +500 from TSS], “stringent” pausing region [TSS to +500], or the gene body/elongating region [+500 to TES])) using the function mergeByOverlaps from the IRanges package. For each gene, the coverage ratios between the pausing regions and the gene body were calculated independently. Mean ratio values across the gene sets of interest were then used as the index values shown in Supplementary Table 6 . Gene functional enrichment analysis and annotation Gene functional enrichments were determined using the DAVID Bioinformatics Resources (v. 6.7) [68] . Annotation clusters identified by DAVID (clusters of related annotation terms) having an enrichment score of ≥1.3 were considered significant and a representative naming for the cluster was derived from the contained Gene Ontology terms. Statistical analysis Lifespan and stress resistance assays were evaluated by Kaplan–Maier and log-rank tests. Statistical analyses for other experiments are stated in the respective methods sections, tables, or figure legends. Analyses were performed using either SPSS (IBM), OASIS [69] , Excel (Microsoft), Graphpad Prism, or R [59] . Reporting summary Further information on research design is available in the Nature Research Reporting Summary linked to this article.